Involvement of the Wnt/β-catenin pathway in neurectoderm architecture inPlatynereis dumerilii Signalling pathways are essential for the correct development of the central nervous system (CNS) in bilaterian animals. Here we show that in the CNS of the annelid Platynereis dumerilii , neural progenitor cells (NPCs) are located close to the ventral midline and express axin , a negative regulator of the Wnt/β-catenin pathway. Using pharmacological inhibitors, we observe that Wnt/β-catenin is required for the transition between proliferating NPCs and differentiating neurons. We also show that the Rho-associated kinase (Rok) is necessary for neurectoderm morphogenesis and ventral midline formation, and indirectly affects the distribution of the NPCs and the development of axonal scaffolds. Moreover, seven genes belonging to the planar cell polarity (PCP) pathway are expressed in the developing Platynereis neurectoderm, suggesting an involvement in its morphogenesis. When compared with previous studies in vertebrates, our data suggest that the involvement of the Wnt/β-catenin pathway in the control of neural cell proliferation/differentiation is ancestral to bilaterians. In bilaterian animals, the architecture of the neurectoderm and the correct development of the central nervous system (CNS) strongly depend on the tightly regulated balance between the renewal of neural progenitor cells (NPCs) and the production of post-mitotic differentiated cells. Whereas this regulation is mainly achieved by intrinsic mechanisms in arthropods such as Drosophila [1] , [2] , in the vertebrate neural tube it crucially depends on long-range signals emanating from dorsal and ventral signalling centres, the roof and floor plates, respectively [3] . In particular, a gradient of Wnt ligands produced by the roof plate stimulates both proliferation [4] , [5] and differentiation of NPCs [6] , [7] in a context-dependent manner, through the activation of the Wnt/β-catenin pathway. Other Wnt molecules, mainly acting through the planar cell polarity (PCP) pathway, also participate in key events of vertebrate CNS development such as neural tube closure [8] , [9] , floor plate formation [10] and axon guidance [11] , [12] . Which aspects of these functions are specific to vertebrates, or ancestral to bilaterians, is still a largely unanswered question owing to the paucity of studies in suitable non-vertebrate models. Over the past decade, the annelid P. dumerilii has become a valuable model for evolutionary developmental biology studies, especially regarding the development of its nervous system that resembles that of vertebrates in many aspects. Studies in Platynereis shed light on several ancestral features of the CNS in bilaterians [13] , including the molecular regionalization of the neurectoderm along the mediolateral axis [14] , the presence of conserved brain neurosecretory cells [15] , and the common ancestry of the vertebrate pallium and the protostome corpora pedunculata [16] . Here, we describe the architecture of the larval neurectoderm in Platynereis and show that the proliferative NPCs are located adjacent to the ventral midline, whereas their differentiating progeny are found in basal/lateral areas. We show that this organization is dependent on the Wnt/β-catenin pathway that is required for the production of neurons by the NPCs. Our data also suggest a signalling role for the ventral midline whose formation depends on a Rho-associated kinase (Rok)-dependent morphogenetic process and might involve the PCP pathway. Cell proliferation in the Platynereis neurectoderm In order to describe the organization and development of the Platynereis neurectoderm, we first revealed the patterns of cell proliferation using 30 min incorporations of 5-ethynyl-2′-deoxyuridine (EdU) at five distinct embryonic stages, ranging from 24 to 72 h post fertilization (hpf) ( Supplementary Fig. S1 ). We observed that between 24 and 33 hpf the neurectoderm consists of only one to two cell layers that are homogenously proliferating ( Fig. 1a–b ). In later stages, the neurectoderm thickens by the addition of cells that do not incorporate EdU in basal and lateral regions, whereas the proliferation area progressively narrows around a thin line of apical ventral midline cells that are themselves non-proliferative ( Fig. 1c–e ). Cells incorporating EdU can also be found in very lateral regions of the ectoderm in a segmentally iterated pattern ( Fig. 1c–e , arrowheads), but their position suggest that they do not belong to the CNS anlagen and rather participate to the development of the epidermis or the peripheral nervous system (PNS). To confirm our EdU data, we isolated several Platynereis cyclin genes ( Supplementary Fig. S2A ) and characterized the expression profile of one of them ( Pdu-cycB-a ) that shows a remarkable similarity to the pattern of EdU incorporation at all studied stages ( Supplementary Fig. S3 ). Cell proliferation profiles were also confirmed by antibody labelling against the phosphorylated form of histone H3 ( Fig. 1f–h ). 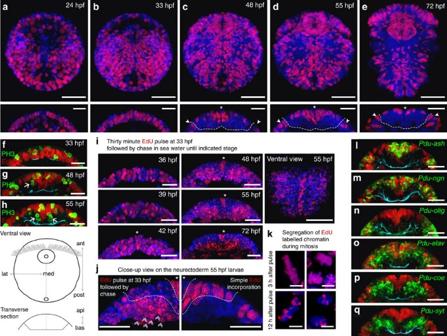Figure 1: Development and architecture of the neurectoderm in the trochophore larvae ofPlatynereis. Ventral views of whole embryos and transverse sections through the neurectoderm are shown. The cartoon in the lower left corner of the figure is shown for orientation purposes. lat, lateral; med, medial; ant, anterior; post, posterior; api, apical; bas, basal. (a–e) Thirty-minute EdU (red) incorporation and Hoechst nuclear staining (blue) at different embryonic stages, showing the reorganization of the cell proliferation profile between 24 and 72 hpf. Dashed lines indicate the limit between the ventral neurectoderm and the lateral ectoderm. (f–h) Thirty-minute EdU incorporation coupled with antibody staining against acetylated tubulin, which marks axon projections in the VNC (cyan), and the phosphorylated form of histone H3 (PH3), which marks cells undergoing mitosis (green). At all studied stages, only a few PH3+ cells could be observed simultaneously, suggesting thatPlatynereis’ neurectodermal cells do not undergo synchronous waves of mitosis, as it is the case for instance inDrosophila, but rather divide independently of each other. Moreover, at 48 and 55 hpf, a few PH3+ cells can be found outside of the area defined by EdU incorporation (arrowheads), suggesting that the external border of the proliferation zone contains cells that will undergo one last division before exiting the cell cycle. (i–k) Pulse and chase experiments involving a 30 min EdU incorporation (red) at 33 hpf followed by chases of various lengths in sea water. These experiments show the formation of distinct cell population after 33 hpf. Asterisks indicate the position of the ventral midline, double arrowheads indicate cells homogenously labelled by EdU and dashed lines demarcate the proliferation zone. (l–q) Simple EdU incorporation (red) on 55 hpf embryos combined with antibody staining against acetylated tubulin (cyan) and WMISH (green) that reveal the expression of several genes involved in the process of neurogenesis. Gene name abbreviations:Pdu-ash,achaete-scute;Pdu-ngn,neurogenin;Pdu-coe,collier;Pdu-syt,synaptotagmin. Scale bars are 50 μm for ventral views, 25 μm for transverse views and 5 μm for high magnification views of dividing cells (k). Figure 1: Development and architecture of the neurectoderm in the trochophore larvae of Platynereis . Ventral views of whole embryos and transverse sections through the neurectoderm are shown. The cartoon in the lower left corner of the figure is shown for orientation purposes. lat, lateral; med, medial; ant, anterior; post, posterior; api, apical; bas, basal. ( a – e ) Thirty-minute EdU (red) incorporation and Hoechst nuclear staining (blue) at different embryonic stages, showing the reorganization of the cell proliferation profile between 24 and 72 hpf. Dashed lines indicate the limit between the ventral neurectoderm and the lateral ectoderm. ( f – h ) Thirty-minute EdU incorporation coupled with antibody staining against acetylated tubulin, which marks axon projections in the VNC (cyan), and the phosphorylated form of histone H3 (PH3), which marks cells undergoing mitosis (green). At all studied stages, only a few PH3+ cells could be observed simultaneously, suggesting that Platynereis ’ neurectodermal cells do not undergo synchronous waves of mitosis, as it is the case for instance in Drosophila , but rather divide independently of each other. Moreover, at 48 and 55 hpf, a few PH3+ cells can be found outside of the area defined by EdU incorporation (arrowheads), suggesting that the external border of the proliferation zone contains cells that will undergo one last division before exiting the cell cycle. ( i – k ) Pulse and chase experiments involving a 30 min EdU incorporation (red) at 33 hpf followed by chases of various lengths in sea water. These experiments show the formation of distinct cell population after 33 hpf. Asterisks indicate the position of the ventral midline, double arrowheads indicate cells homogenously labelled by EdU and dashed lines demarcate the proliferation zone. ( l – q ) Simple EdU incorporation (red) on 55 hpf embryos combined with antibody staining against acetylated tubulin (cyan) and WMISH (green) that reveal the expression of several genes involved in the process of neurogenesis. Gene name abbreviations: Pdu-ash , achaete-scute ; Pdu-ngn , neurogenin ; Pdu-coe , collier ; Pdu-syt , synaptotagmin . Scale bars are 50 μm for ventral views, 25 μm for transverse views and 5 μm for high magnification views of dividing cells ( k ). Full size image We next estimated the contribution of the 33 hpf proliferative cells to the development of the neurectoderm by performing a 30 min pulse of EdU at 33 hpf followed by chases in sea water. After 3–9 h chases, we observed that a great majority of neurectodermal cells displayed a strong and homogenous EdU labelling ( Fig. 1i ). After 15 h or longer chases, we could distinguish several populations of cells based on position and EdU labelling ( Fig. 1i ). One of them is the ventral midline that occupies a medial and apical position, extends along the anterior–posterior axis of the embryo and consists of a continuous row of one to two cells that are homogenously labelled by EdU ( Fig. 1i , 48 to 72 hpf, asterisks). Other homogenously labelled cells were found in the most basal layers of the neurectoderm ( Fig. 1j , left panel, double arrowheads), whereas cells occupying intermediate layers showed a much weaker and stippled labelling. A comparison with embryos that were incubated with EdU for 30 min at 55 hpf ( Fig. 1j , right panel) revealed that the cells that show the weakest labelling after a 22 h chase are actually proliferating cells surrounding the ventral midline. We analysed the dynamics of EdU-labelled chromatin during cell division by looking at mitotic figures after short or long chases following EdU incorporation in 33 hpf larvae ( Fig. 1k ). These observations suggest that, during pulse and chase experiments, cells that did not divide or divided a very limited number of times show a homogenous EdU labelling, whereas cells that went through multiple rounds of division show a very weak and stippled labelling, thus giving information about the order in which the different cell populations were produced. We conclude that, from the cells that were proliferating at 33 hpf, few of them rapidly exited the cell cycle, and gave rise to the apical ventral midline and the most basal layers of the neurectoderm. Other post-mitotic layers were formed afterwards through more divisions. Finally, active proliferation is maintained in cells located in the vicinity of the ventral midline, which explains their extremely weak and stippled EdU labelling during pulse and chase experiments. Architecture of the developing neurectoderm in Platynereis We next combined EdU incorporations with whole mount in situ hybridization (WMISH) on 55 hpf embryos to correlate the expression of known marker genes for specific steps of neurogenesis [14] , [17] , [18] , [19] with the different cell populations defined in the previous experiments. First we found that the proneural genes achaete-scute ( Pdu-ash ) and neurogenin ( Pdu-ngn ) are exclusively expressed in proliferating cells ( Fig. 1l ), suggesting that these cells are NPCs. Additionally Pdu-olig , another NPCs gene that marks PNS cells in Platynereis (unpublished observations), is only expressed in the most lateral proliferative cells ( Fig. 1n ). We therefore conclude that at least two populations of NPCs are present in the ectoderm of 55 hpf larvae: on one hand, PNS progenitors that express Pdu-ash , Pdu-ngn , and Pdu-olig ; on the other hand, neural progenitors of the CNS that surround the ventral midline and express Pdu-ash and Pdu-ngn . We also compared the pattern of EdU incorporation with the expression profiles of Pdu-elav , a well-known marker of the switch between NPCs proliferation and differentiation, and two markers of neuronal differentiation, collier ( Pdu-coe ) and synaptotagmin ( Pdu-syt ). We observed Pdu-elav expression in both post-mitotic cells and in some of the proliferating cells that also express Pdu-ngn ( Fig. 1o ), whereas Pdu-coe and Pdu-syt are exclusively expressed in cells that do not incorporate EdU ( Fig. 1p ). We therefore identified these cells as differentiating and/or fully differentiated neurons. Based on cell proliferation assays and WMISH, we conclude that Platynereis ’ neurectoderm is composed of multiple layers, each containing cells at a defined step of the neurogenesis process. These cell layers are organized around the apically located ventral midline and occupy defined positions along both the apicobasal and mediolateral axes ( Supplementary Fig. S4 ). Proliferating NPCs of the CNS are found in the vicinity of the ventral midline, whereas differentiating neurons populate the more basal and lateral areas. We next looked for signalling pathways that may be involved in setting up this architecture. Given its major involvement in the control of cell proliferation and differentiation in the vertebrate CNS [4] , [5] , [6] , [7] , we focused on the Wnt/β-catenin pathway. Expression of Wnt/β-catenin pathway genes in neurectoderm Among the 12 genes encoding Wnt ligands identified in Platynereis [20] , one of them, Pdu-wnt4 , is expressed at 33 hpf in a single stripe that runs across the ventral ectoderm, and at 55 hpf both in ventral midline cells and segmental stripes restricted to the lateral ectoderm ( Fig. 2a ). To define whether a Wnt/β-catenin pathway is active in the Platynereis neurectoderm, we cloned Pdu-wntless ( Supplementary Fig. S2B ), which encodes a cargo protein responsible for the transport and secretion of Wnt ligands [21] , [22] , and Pdu-axin ( Supplementary Fig. S2C ), a key protein of the β-catenin degradation complex [23] , [24] . At 33 hpf Pdu-wntless is weakly expressed in a few neurectodermal cells ( Fig. 2b ), but at 55 hpf its expression is observed both in the medial region of the neurectoderm and in the lateral ectoderm ( Fig. 2b ). Pdu-axin is expressed in two bilateral longitudinal domains in the neurectoderm at 33 hpf ( Fig. 2c ), and then in the proliferating cells that surround the ventral midline at 55 hpf ( Fig. 2c ). The expression of members of the Wnt/β-catenin pathway in restricted regions of the neurectoderm at the time the organization of cell proliferation and differentiation is set up (33 to 55 hpf) is therefore suggestive of an involvement of the pathway in the establishment of the architecture of the Platynereis neurectoderm. 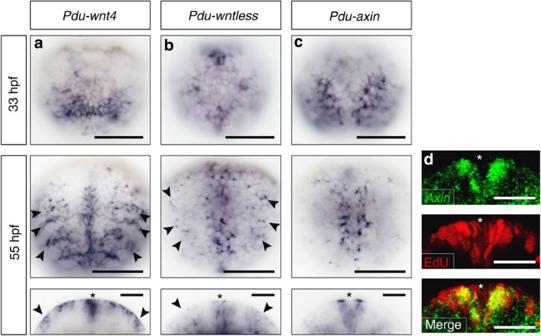Figure 2: Expression patterns of threePlatynereisgenes encoding members of the Wnt/b-catenin pathway. Ventral views of whole embryos and transverse sections through the neurectoderm are shown. See the cartoon inFig. 1for orientations. (a–c) WMISH showing thatPdu-wnt4,Pdu-wntlessandPdu-axinare expressed in the neurectoderm of 33 hpf and 55 hpf larvae. Arrowheads indicate the expression ofPdu-wnt4andPdu-wntlessin lateral ectodermal cells. Asterisks indicate the position of the ventral midline on transverse sections. (d) Thirty-minute EdU incorporation (red) coupled with WMISH forPdu-axin(green) shows that the gene is expressed in proliferating cells at 55 hpf. Scale bars are 50 μm for ventral views and 25 μm for transverse views. Figure 2: Expression patterns of three Platynereis genes encoding members of the Wnt/b-catenin pathway. Ventral views of whole embryos and transverse sections through the neurectoderm are shown. See the cartoon in Fig. 1 for orientations. ( a – c ) WMISH showing that Pdu-wnt4 , Pdu-wntless and Pdu-axin are expressed in the neurectoderm of 33 hpf and 55 hpf larvae. Arrowheads indicate the expression of Pdu-wnt4 and Pdu-wntless in lateral ectodermal cells. Asterisks indicate the position of the ventral midline on transverse sections. ( d ) Thirty-minute EdU incorporation (red) coupled with WMISH for Pdu-axin (green) shows that the gene is expressed in proliferating cells at 55 hpf. Scale bars are 50 μm for ventral views and 25 μm for transverse views. Full size image Wnt/b-catenin regulates NPC proliferation vs differentiation In order to test this hypothesis, we performed in vivo treatments using cell permeable small molecule inhibitors of the Wnt/β-catenin pathway, endo-IWR-1 [25] and PNU-74654 [26] . Endo-IWR-1 acts as a stabilizer of Axin, thereby stimulating the degradation of cytoplasmic β-catenin and constitutively inhibiting the Wnt/β-catenin pathway, without altering the pool of membrane tethered β-catenin [25] , [27] . This molecule has been shown to reduce the amount of β-catenin and to inhibit the transcriptional response to Wnt/β-catenin signalling in developing zebrafish and Xenopus embryos and larvae [28] , [29] , indicating its suitability for in vivo studies. In order to confirm endo-IWR-1 phenotypes, we used PNU-74654 that prevents the interaction between β-catenin and the transcription factor TCF [26] , [30] . Treatment with either molecule from 33 to 55 hpf allowed us to avoid interferences with earlier global functions of β-catenin [31] , and to specifically target the period during which cell proliferation reorganizes around the ventral midline and massive neural differentiation occurs. Effects of the treatments were analysed using 30 min EdU incorporation at 55 hpf and antibody labelling against acetylated tubulin to reveal the axonal scaffold of the ventral nerve cord (VNC). Very similar effects were observed with the two inhibitors that target two different members of the Wnt/β-catenin pathway ( Fig. 3 and Supplementary Fig. S5 ), corroborating the specificity and validity of the used molecules to inhibit this pathway. We tried to demonstrate an effect of the two small molecules on β-catenin localization or degradation, using an antibody against vertebrate β-catenin, which previously allowed to detect nuclear β-catenin in very early stages of Platynereis development [31] , and a newly developed antibody against the Platynereis protein (unpublished). We failed to detect any nuclear β-catenin labelling in 33 hpf and 55 hpf embryos (not shown), precluding the use of the antibodies to visualize the activation of the Wnt/β-catenin pathway and the effect of the small molecules on the pathway. 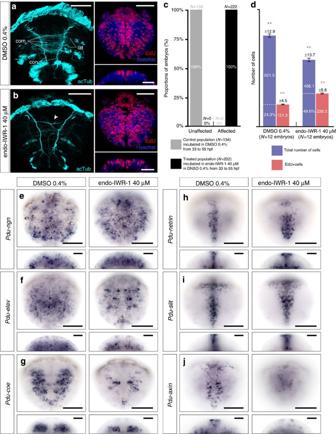Figure 3: Inhibition of the Wnt/b-catenin pathway induces defects in CNS formation. Ventral views of whole embryos and transverse sections through the neurectoderm are shown. See the cartoon inFig. 1for orientations. Embryos were incubated with endo-IWR-1 (40 μM) in DMSO (0.4%) or in DMSO only (control group) from 33 to 55 hpf. (a–b) Antibody labelling against acetylated tubulin (cyan) showing the axon scaffold of the VNC, coupled with 30 min EdU (red) incorporation at 55 hpf showing the cell proliferation profile and Hoechst nuclear staining (blue). Embryos treated with endo-IWR-1 display a clear reduction of the axonal tracts of the VNC, defects in axon guidance (arrowhead) and an extension of the cell proliferation profile. Abbreviations: con, longitudinal connectives; com, commissural axons; lat, lateral projections. (c) Graph showing the proportions of affected versus unaffected embryos in the control and treated groups (sample sizes are indicated on the graph). The experiment was replicated three times. All control embryos are unaffected and all treated embryos are affected. (d) Graph showing the total amount of cells (Hoechst+, blue) and the amount of proliferating cells (EdU+, red) in the neurectoderm of 12 control and 12 treated embryos. Values indicate the mean±s.e.m. The percentages of CNS cells that are labelled by EdU are also indicated. Blue asterisks indicate a significant difference between the mean number of Hoechst-labelled cells in control and treated embryos (Student’st-test,P=1.17 × 10−8,n=12). Red asterisks indicate a significant difference between the mean number of EdU-labelled cells in control and treated embryos (Student’st-test,P=5.16 × 10−10,n=12). (e–j) WMISH revealing the expression of several genes involved in the process of neurogenesis in control and treated embryos. Gene name abbreviations:Pdu-ngn,neurogenin;Pdu-coe,collier. Scale bars are 50 μm for ventral views and 25 μm for transverse views. Figure 3: Inhibition of the Wnt/b-catenin pathway induces defects in CNS formation. Ventral views of whole embryos and transverse sections through the neurectoderm are shown. See the cartoon in Fig. 1 for orientations. Embryos were incubated with endo-IWR-1 (40 μM) in DMSO (0.4%) or in DMSO only (control group) from 33 to 55 hpf. ( a – b ) Antibody labelling against acetylated tubulin (cyan) showing the axon scaffold of the VNC, coupled with 30 min EdU (red) incorporation at 55 hpf showing the cell proliferation profile and Hoechst nuclear staining (blue). Embryos treated with endo-IWR-1 display a clear reduction of the axonal tracts of the VNC, defects in axon guidance (arrowhead) and an extension of the cell proliferation profile. Abbreviations: con, longitudinal connectives; com, commissural axons; lat, lateral projections. ( c ) Graph showing the proportions of affected versus unaffected embryos in the control and treated groups (sample sizes are indicated on the graph). The experiment was replicated three times. All control embryos are unaffected and all treated embryos are affected. ( d ) Graph showing the total amount of cells (Hoechst+, blue) and the amount of proliferating cells (EdU+, red) in the neurectoderm of 12 control and 12 treated embryos. Values indicate the mean±s.e.m. The percentages of CNS cells that are labelled by EdU are also indicated. Blue asterisks indicate a significant difference between the mean number of Hoechst-labelled cells in control and treated embryos (Student’s t -test, P =1.17 × 10 −8 , n =12). Red asterisks indicate a significant difference between the mean number of EdU-labelled cells in control and treated embryos (Student’s t -test, P =5.16 × 10 −10 , n =12). ( e – j ) WMISH revealing the expression of several genes involved in the process of neurogenesis in control and treated embryos. Gene name abbreviations: Pdu-ngn , neurogenin ; Pdu-coe , collier . Scale bars are 50 μm for ventral views and 25 μm for transverse views. Full size image In comparison with dimethylsulphoxide (DMSO)-incubated control embryos that appear unaffected ( Fig. 3a ), all endo-IWR-1-treated animals displayed a marked alteration of the VNC, with a strongly reduced number of lateral and commissural projections, as well as defects in axon guidance ( Fig. 3b arrowhead, c). We also observed the presence of proliferating cells scattered across the whole neurectoderm of treated embryos ( Fig. 3b ), whereas in the control group these cells are found only in the vicinity of the ventral midline and in peripheral regions ( Fig. 3a ). To determine if this disorganization is owing to an increase in the number of proliferating cells or solely to their dispersal, we quantified EdU-labelled cells ( Fig. 3d ) and found a significantly higher number of proliferative cells in treated embryos compared with the control, indicating that the endo-IWR-1 treatment led to increased cell proliferation. We also observed that the total number of cells in the CNS (defined by quantifying Hoechst-labelled cells) is significantly smaller in treated embryos than in controls ( Fig. 3d ). To define whether this could be owing to endo-IWR-1-induced cell death, we established a terminal deoxynucleotidyl transferase dUTP nick end labelling (TUNEL) protocol for Platynereis and found an absence of apoptotic cells in the neurectoderm of treated embryos ( Supplementary Fig. S6 ). We thus suggest that the reduction in the total number of CNS cells is owing to the fact that no or very few differentiated neural cells were produced during the time of exposure to endo-IWR-1. These data therefore strongly suggest that Wnt/β-catenin inhibition blocks neurectodermal cells in a proliferative state and impairs the production of differentiated cells. We further characterized the phenotype by performing a series of WMISH for several genes involved in the neurogenesis process in Platynereis on control and endo-IWR-1-treated embryos. We found expression of the proliferating NPCs marker Pdu-ngn in most layers of the neurectoderm in treated embryos, whereas in control animals expression of this gene is only found in cells close to the ventral midline ( Fig. 3e ). Consistent with the increased number of EdU-labelled cells, this suggests that the inhibition of the Wnt/βcatenin pathway leads to an increase in the number of proliferative NPCs. Conversely, endo-IWR-1 strongly reduces the amount of neurons, as seen by the loss of many Pdu-elav - and Pdu-coe -expressing cells in treated embryos ( Fig. 3f ), suggesting that the Wnt/β-catenin pathway is required for neuron formation in Platynereis . This failure in the production of neurons would explain the reduction of both the axonal scaffolds ( Fig. 3b ) and the number of CNS cells ( Fig. 3d ) in the endo-IWR-1-treated embryos. We also found that the expression domains of the ventral midline markers Pdu-slit , and Pdu-netrin [14] , are slightly enlarged in treated embryos ( Fig. 3h–i ), suggesting that the endo-IWR-1 treatment might interfere with ventral midline formation. By analogy to the known roles of slit and netrin during axon guidance in the CNS of vertebrates and arthropods [32] , mild defects in ventral midline formation might explain the axon guidance defects that we observed in endo-IWR-1-treated embryos. Finally, we observed that Pdu-axin expression is strongly reduced in endo-IWR-1-treated embryos ( Fig. 3j ), suggesting that, like in vertebrates [33] , [34] , [35] , axin expression is dependent on Wnt/β-catenin pathway activity in Platynereis . This latter conclusion is reinforced by the observation of a very strong increase in the expression of Pdu-axin in embryos treated with azakenpaullone, an inhibitor of glycogen synthase kinase-3 that constitutively activates the Wnt/β-catenin pathway [31] , [36] , [37] ( Supplementary Fig. S7 ). Taken together, our results suggest that the Wnt/β-catenin pathway, whose function involves an axin -based negative feedback loop, is required for neuron production in the Platynereis CNS and regulates the transition between proliferating NPCs and post-mitotic differentiating cells. CNS development requires Rok-dependent midline formation Our data regarding the architecture of the neurectoderm, the expression profiles of genes such as Pdu-wnt4 , Pdu-slit and Pdu-netrin , and the function of the Wnt/β-catenin pathway suggest that the ventral midline may act as an organizing centre, which produces signals important for neuron production and the proper scaffolding of the VNC. Ventral midline formation depends on the medial fusion of the left and right halves of the neurectoderm that occurs during the 24 to 33 hpf period [14] . To test the possible roles of the ventral midline in CNS development, we tried to prevent or alter its formation, using Y-27632 [38] , [39] , a highly specific inhibitor of Rok that has been shown to impair morphogenetic movements involved in neural tube closure and floor plate formation in zebrafish embryos [40] , [41] . Both Rok and its associated GTPase RhoA ( Supplementary Fig. S2G,I ) are ubiquitously expressed in the whole ectoderm of Platynereis embryos (not shown). Embryos treated with Y-27632 from 24 to 33 hpf and then placed in sea water until 55 hpf show a range of defects in the axonal scaffolds of their CNS, their EdU incorporation profile, and the morphology of their neurectoderm ( Fig. 4a–e ). Similar defects were observed with a longer treatment (24–55 hpf), whereas most embryos treated from 33 to 55 hpf were unaffected or showed very mild defects ( Fig. 4e ). This suggests that most of the effects of the treatment were caused by the inhibition of Rok function between 24 and 33 hpf. Interestingly, the most affected embryos in terms of axonal defects and disorganized EdU incorporation profile (class 3; Fig. 4d ) also show the presence of a gap in the middle of the neurectoderm, indicating that the fusion of the two halves of the neurectoderm was not properly achieved. WMISH for Pdu-ngn , Pdu-elav and Pdu-coe revealed that, although the distribution of NPCs is abnormal in embryos treated with Y-27632, many neurons are produced, even in class 3 embryos ( Fig. 4f–h ). This suggests that Rok is not required for neuron differentiation, and that the lack of axon projections is solely owing to defects in neuron terminal differentiation and/or axon growth or guidance. We also observed that ventral midline markers are still expressed in Y-27632-treated embryos, even though in class 3 embryos, their expression domains are split into two symmetric populations of cells occupying the medial borders of the opened neurectoderm ( Fig. 4i–j ). A slight disorganization and/or enlargement of these same expression domains were also observed in less affected embryos (class 2, Fig. 4i–j ), suggesting that the Y-27632 treatment interferes with proper ventral midline organization, even in cases where the medial fusion of the neurectoderm actually occurred. 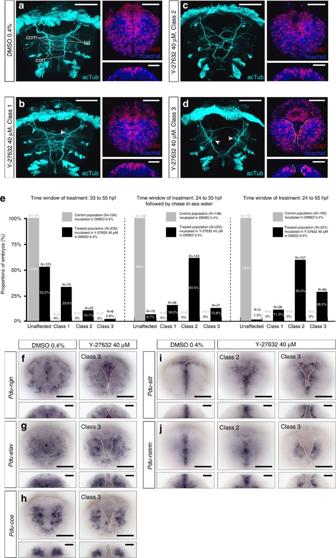Figure 4: Inhibition of Rok activity causes defects in neurectoderm architecture and axon guidance. Ventral views of whole embryos and transverse sections through the neurectoderm are shown. See the cartoon inFig. 1for orientations. Embryos were incubated with Y-27632 (40 μM) in DMSO (0.4%) or in DMSO only (control group) during three different time windows: from 24 to 33 hpf (followed by chase in sea water until 55 hpf); from 33 to 55 hpf; or from 24 to 55 hpf. (a–d) Antibody labelling against acetylated tubulin (cyan) and 30 min EdU (red) incorporation at 55 hpf were analysed and allowed to define four phenotypical classes. (a) Control embryos are normal. (b) Class1 embryos show a few defects in axon guidance and a slight disorganization of the EdU incorporation profile. (c) Class 2 embryos display a loss of commissural projections, severe defects in axon guidance and an altered EdU incorporation profile. (d) Class 3 embryos show abnormally moved apart connectives, an extreme loss of axon projections, a disorganized EdU incorporation profile and the presence of a gap in the middle of the neurectoderm. con, longitudinal connectives; com, commissural axons; lat, lateral projections. (e) Graph showing the proportions of affected versus unaffected embryos in the control and treated groups, depending on the time window of the treatment (sample sizes are indicated on the graph). The experiment was replicated three times. Control embryos incubated with DMSO were all unaffected. Most embryos treated from 33 to 55 hpf were unaffected (53.2%) or belonged to class 1 (33.6%). A majority of embryos treated from 24 to 33 hpf, or from 24 to 55 hpf, belonged to class 2 (63.5% and 59.3%, respectively) and to a lesser extent to class 3 (13.8% and 28.2%, respectively). (f–j) WMISH revealing the expression of several genes involved in the process of neurogenesis. Gene name abbreviations:Pdu-ngn,neurogenin;Pdu-coe,collier. White dotted lines indicate the borders of the blastopore in class 3 embryos, in which the neurectoderm is abnormally opened. Class 2 embryos were recognized as such based on their frequency in the treated population. Scale bars are 50 μm for ventral views and 25 μm for transverse views. Figure 4: Inhibition of Rok activity causes defects in neurectoderm architecture and axon guidance. Ventral views of whole embryos and transverse sections through the neurectoderm are shown. See the cartoon in Fig. 1 for orientations. Embryos were incubated with Y-27632 (40 μM) in DMSO (0.4%) or in DMSO only (control group) during three different time windows: from 24 to 33 hpf (followed by chase in sea water until 55 hpf); from 33 to 55 hpf; or from 24 to 55 hpf. ( a – d ) Antibody labelling against acetylated tubulin (cyan) and 30 min EdU (red) incorporation at 55 hpf were analysed and allowed to define four phenotypical classes. ( a ) Control embryos are normal. ( b ) Class1 embryos show a few defects in axon guidance and a slight disorganization of the EdU incorporation profile. ( c ) Class 2 embryos display a loss of commissural projections, severe defects in axon guidance and an altered EdU incorporation profile. ( d ) Class 3 embryos show abnormally moved apart connectives, an extreme loss of axon projections, a disorganized EdU incorporation profile and the presence of a gap in the middle of the neurectoderm. con, longitudinal connectives; com, commissural axons; lat, lateral projections. ( e ) Graph showing the proportions of affected versus unaffected embryos in the control and treated groups, depending on the time window of the treatment (sample sizes are indicated on the graph). The experiment was replicated three times. Control embryos incubated with DMSO were all unaffected. Most embryos treated from 33 to 55 hpf were unaffected (53.2%) or belonged to class 1 (33.6%). A majority of embryos treated from 24 to 33 hpf, or from 24 to 55 hpf, belonged to class 2 (63.5% and 59.3%, respectively) and to a lesser extent to class 3 (13.8% and 28.2%, respectively). ( f – j ) WMISH revealing the expression of several genes involved in the process of neurogenesis. Gene name abbreviations: Pdu-ngn , neurogenin ; Pdu-coe , collier . White dotted lines indicate the borders of the blastopore in class 3 embryos, in which the neurectoderm is abnormally opened. Class 2 embryos were recognized as such based on their frequency in the treated population. Scale bars are 50 μm for ventral views and 25 μm for transverse views. Full size image We conclude that Rok is involved in the morphogenetic process that leads to the fusion of the neurectoderm after 24 hpf and to the formation of the neural ventral midline. Impairment of neurectoderm fusion and midline formation observed upon Rok inhibition indirectly causes an abnormal NPCs distribution and important defects in the axonal scaffold of the VNC. These observations therefore support the hypothesis of a signalling role of the ventral midline during Platynereis CNS development. Rok might act downstream of PCP signalling In many vertebrate morphogenetic processes, Rok has been shown to act as an effector of the PCP pathway [40] , [41] , [42] , [43] , [44] . We therefore isolated and characterized the expression patterns of several genes encoding members of the PCP pathway in Platynereis . The global module of the PCP pathway includes the atypical cadherins Fat and Dachsous (Ds), and their regulator Four-jointed (Fj), a Golgi-associated kinase [45] , [46] . This module establishes a polarity at the scale of the tissue via the opposite transcriptional gradients of ds and fj [45] , [46] . Highly reminiscent of this situation, Platynereis ds and fj ( Supplementary Fig. S2J–L ) are expressed in the neurectoderm at 33 and 55 hpf ( Fig. 5a–b ) in two opposite gradients along the mediolateral axis. In contrast, Pdu-fat expression is broad in the neurectoderm at 33 hpf and restricts to ventral midline cells by 55 hpf ( Fig. 3c ). These data suggest that the ventral neurectoderm of Platynereis is polarized via the Fat–Ds–Fj system along the mediolateral axis. The core PCP module, which relays the global polarity of the tissue at the cellular level, includes flamingo/starrynight / celsr and Vangogh/strabismsus , which encode transmembrane proteins, as well as Prickle and diego/inversin , which encode cytoplasmic proteins [45] , [47] . Most of these genes are required for neurulation in the developing vertebrate CNS [8] , [10] , [48] . In Platynereis , Pdu-flamingo , Pdu-stbm [49] , Pdu-prickle and Pdu-diego ( Supplementary Fig. S2D–F ) are broadly expressed in the neurectoderm at 33 hpf ( Fig. 5d–g ), whereas at 55 hpf their expression becomes restricted in the cells that surround the ventral midline ( Fig. 5d–g ). 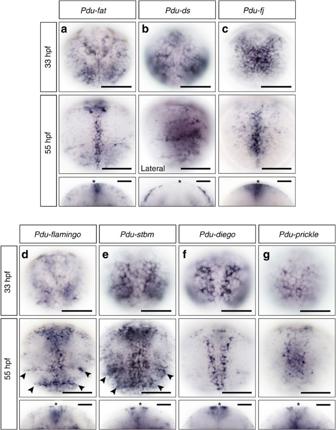Figure 5: Expression patterns of sevenPlatynereisgenes encoding members of the PCP pathway. Ventral views of whole embryos (unless mentioned otherwise) and transverse sections through the neurectoderm are shown. See the cartoon inFig. 1for orientations. (a–c) WMISH ofPdu-fat,Pdu-dsandPdu-fj, which encode members of the global PCP module and are expressed in the neurectoderm at 33 and 55 hpf.Pdu-dsandPdu-fjdisplay opposite gradients of expression along the mediolateral axis. (d–g) WMISH ofPdu-flamingo,Pdu-stbm,Pdu-diegoandPdu-prickle, which encode members of the core PCP module and are all expressed in the neurectoderm at 33 hpf, although very weakly forPdu-flamingoandPdu-prickle. At 55 hpf, the four genes are expressed in the proliferating NPCs that surround the ventral midline. Arrowheads indicate posterior and lateral areas ofPdu-flamingoandPdu-stbmexpression that may correspond to segmental stripes. Asterisks indicate the position of the ventral midline on transverse sections. Gene name abbreviations:Pdu-ds,dachsous;Pdu-fj,four-jointed;Pdu-stbm,strabismus. Scale bars are 50 μm for ventral views and 25 μm for transverse views. Figure 5: Expression patterns of seven Platynereis genes encoding members of the PCP pathway. Ventral views of whole embryos (unless mentioned otherwise) and transverse sections through the neurectoderm are shown. See the cartoon in Fig. 1 for orientations. ( a – c ) WMISH of Pdu-fat , Pdu-ds and Pdu-fj , which encode members of the global PCP module and are expressed in the neurectoderm at 33 and 55 hpf. Pdu-ds and Pdu-fj display opposite gradients of expression along the mediolateral axis. ( d – g ) WMISH of Pdu-flamingo , Pdu-stbm , Pdu-diego and Pdu-prickle , which encode members of the core PCP module and are all expressed in the neurectoderm at 33 hpf, although very weakly for Pdu-flamingo and Pdu-prickle . At 55 hpf, the four genes are expressed in the proliferating NPCs that surround the ventral midline. Arrowheads indicate posterior and lateral areas of Pdu-flamingo and Pdu-stbm expression that may correspond to segmental stripes. Asterisks indicate the position of the ventral midline on transverse sections. Gene name abbreviations: Pdu-ds , dachsous ; Pdu-fj , four-jointed ; Pdu-stbm , strabismus . Scale bars are 50 μm for ventral views and 25 μm for transverse views. Full size image Our data therefore indicate that several genes of the PCP pathway are expressed in restricted domains along the mediolateral axis of the neurectoderm, suggesting that the pathway is active during neurectoderm development and that, like in vertebrates, Rok may act as an effector of the PCP pathway in CNS morphogenesis. Our detailed study of the architecture of the Platynereis neurectoderm at 55 hpf indicates that proliferating NPCs occupy apical and medial positions close to the ventral midline, whereas post-mitotic differentiating neurons are found in more basal and lateral areas ( Supplementary Fig. S4 ). This organization is established from 33 hpf and afterwards, concomitantly with the differentiation of the ventral midline and involves the Wnt/β-catenin pathway. We show that Pdu-axin , a negative regulator of the Wnt/β-catenin pathway, is specifically expressed in the proliferating NPCs of the CNS ( Fig. 2d ). Stabilization of Axin protein through endo-IWR-1 treatment leads to a loss of neurons and an increase in the number of proliferating NPCs ( Fig. 3 ). Similar effects were obtained with an unrelated inhibitor of the Wnt/β-catenin pathway, PNU-74654, which prevents the interaction between β-catenin and TCF ( Supplementary Fig. S5 ). Our results therefore indicate that the Wnt/β-catenin pathway is required for the transition from proliferative NPCs towards post-mitotic differentiating cells in the Platynereis CNS. A similar requirement of the Wnt/β-catenin pathway for neuron differentiation has been shown in vertebrates [6] , [7] . Whether the pathway may also promote neural cell proliferation like in vertebrates [4] , [5] at other stages and/or other parts of the nervous system in Platynereis (for example, brain or PNS) remains to be determined. Our results also show that the expression of Pdu-axin is dependent on the Wnt/β-catenin pathway: its expression is strongly decreased in embryos treated with inhibitors of the pathway (endo-IWR-1 and PNU-74654; Fig. 3 and Supplementary Fig. S5 ) and strongly increased in embryos treated with azakenpaullone, an activator of the pathway ( Supplementary Fig. S7 ). This is similar to what has been observed in vertebrates, in which axin2 is a transcriptional target of the Wnt/β-catenin pathway in many tissues [33] , and suggests that a negative feedback loop involving axin participates in the regulation of the Wnt/β-catenin pathway activity in the Platynereis neurectoderm. Given that Pdu-wnt4 is the only Platynereis wnt gene expressed by ventral midline cells [20] and that Pdu-axin is only expressed in the cells that are located very close to the ventral midline, we suggest that a Wnt4 signal emanating from the ventral midline cells would be responsible for the activation of Pdu-axin expression. This assumption is reinforced by the expression in midline cells of Pdu-Wntless/Evi whose orthologues are required for Wnt protein secretion [21] , [22] . Our working model is therefore that a short-range Pdu-Wnt4 signal would have two opposite effects. First, it would stimulate some NPCs to exit from the cell cycle and to enter a differentiation programme, thereby allowing the production of neurons. Then, through the activation of Pdu-axin expression, it would also allow other NPCs to be ‘protected’ from the differentiation signal and to remain in a proliferative state. An interesting observation is that Pdu-axin is only strongly expressed in the proliferating cells that are the closest to the ventral midline, and not or very weakly in those that are more distant from the midline ( Fig. 2d ). This would be consistent with a dosage-dependent model in which cells close to the midline receive a strong Wnt signal that activates Pdu-axin expression, whereas cells located further away would receive a weaker signal sufficient to stimulate differentiation but not to activate Pdu-axin expression. The expression of Pdu-Wnt4 in Platynereis ventral midline cells is similar to the expression of vertebrate Wnt4 genes in the floor plate [4] , [50] , [51] . The floor plate corresponds to the vertebrate CNS dorsal midline and is thought to be homologous to the Platynereis ventral midline [13] , [14] , therefore pointing out a deep evolutionary conservation of the expression of wnt4 genes in bilaterians. However, floor plate-secreted Wnt4 proteins are not involved in the control of cell proliferation and differentiation in the vertebrate neural tube and instead have been shown to control the antero–posterior guidance of commissural axons [50] , as well as some other unrelated processes such as segmental patterning [51] and midline convergence of organ primordia [52] . By controlling neural cell differentiation and proliferation, ventral midline-secreted Pdu-Wnt4 would therefore have a strikingly different function than its vertebrate homologue, and would be functionally comparable to the vertebrate Wnt1 and Wnt3a produced by the roof plate of the neural tube [4] . If the involvement of the Wnt/β-catenin pathway in the regulation of neural cells proliferation versus differentiation is ancestral to bilaterians, the question of the identity and localization of the Wnt signal that exerted this function in their last common ancestor remains opened. Rok pathway inhibition, using the Y-27632 small molecule, reinforces the hypothesis of a signalling role of the ventral midline. Indeed, we observed that an early treatment (24 to 33 hpf) with this inhibitor indirectly alters the distribution of neural progenitors at later stages (55 hpf), most likely owing to the effect of Rok inhibition on the formation of the ventral midline. While the role of Platynereis ’ ventral midline still requires experimental demonstration, for instance through the production of embryos depleted of midline cells, it is in concordance with existing data that show an organizing role of the midline in vertebrates [53] and in the arthropod Parhyale hawaiensis [54] , suggesting that the existence of a CNS midline with a signalling activity might be a conserved feature in bilaterians. Gene cloning and identification Platynereis genes were identified by sequence similarity searches against a large collection of expressed sequence tags (ESTs) and genomic sequences [55] using Drosophila and/or vertebrate genes as query. Gene fragments were subsequently cloned using PCR on complementary DNAs from mixed larval stages (primer sequences can be found below). The predicted amino-acid sequences of the identified Platynereis gene fragments were aligned with their presumptive orthologues from a selection of animal groups. These genes were either annotated as such in public databases, or found as predicted genes in whole-genome BLAST screening. Multiple alignments were performed with MUSCLE 3.7 (ref. 56 ) using the Phylogeny.fr web server and were subsequently manually improved. Maximum likelihood analyses were performed using PHYML [57] with the Le and Gascuel amino-acid substitution model and two rate categories (one constant and four gamma rates). Statistical support for the different internal branches was assessed by approximate Likelihood-ratio test. The whole list of sequences used in this study and the multiple alignments are available upon request. PCR primers Primers are listed in the same order as the corresponding genes appear in the main text. Pdu-cyclin B-a forward primer: 5′-GAAACACTGAACACAACGAACGAAT-3′; Pdu-cyclin B-a reverse primer: 5′-GAGGTCCGTTATGAGATCGCTT-3′; Pdu-cyclin B-b forward primer: 5′-CGTCCGCTCAACTTATCACA-3′; Pdu-cyclin B-b reverse primer: 5′-CTTCATAGGAGGGGCAAGG-3′; Pdu-cyclin 3 forward primer: 5′-CAGCTAAAGCGTCGTTGTGA-3′; Pdu-cyclin 3 reverse primer: 5′-ACAAAATGGAGGGAGGCATT-3′; Pdu-wntless forward primer: 5′-CGCAACATCAGTGCCAGCGAGATTG-3′; Pdu-wntless reverse primer: 5′-TGCGACTCATACTGATCTAGAAGCT-3′; Pdu-axin forward primer: 5′-TCAGAAGTTCCTCAATGACTCG-3′; Pdu-axin reverse primer: 5′-GTCTGACCCCAGAATTGTC-3′; Pdu-flamingo forward primer: 5′-GTACCATTTGGATAAGTTGAAAAG-3′; Pdu-flamingo reverse primer: 5′-CGTTATCGTTGACATCAATCACTCG-3′; Pdu-diego forward primer: 5′-CGGTTACACAGCTCTCCACA-3′; Pdu-diego reverse primer: 5′-ACCAGCAGTTGTTCCCACTC-3′; Pdu-prickle forward primer: 5′-AACCTGGACCACGATGAGAT-3′; Pdu-prickle reverse primer: 5′-TTTCGGCATGATGTCTACCA-3′; Pdu-rho forward primer: 5′-TCCGTCTGACTGGTCGGTCAAAGA-3′; Pdu-rho reverse primer: 5′-ATCACTAAGATGACTACACAACGAG-3′; Pdu-rac forward primer: 5′-CGTCCGCCATTTTGACTACAAGGCA-3′; Pdu-rac reverse primer: 5′-TCTGTAATCACATCTCTATACAAAT-3′; Pdu-rok forward primer: 5′-GGTCTGTAGGGGTATTTCTCTATG-3′; Pdu-rok reverse primer: 5′-CCTTGTGACTTGGCATTTTGCTC-3′; Pdu-four-jointed forward primer: 5′-GGAGGCACTGCTAGCCAGACACTAG-3′; Pdu-four-jointed reverse primer: 5′-ATTGTTAATTGAACGACTCGATCAC-3′; Pdu-fat forward primer: 5′-ATGACAACAGACCGGCCTTC-3′; Pdu-fat reverse primer: 5′-CTTTCGCAGACACGTTGAGG-3′; Pdu-dachsous forward primer: 5′-GAGCGGCACCTTTGATATGTC-3′; Pdu-dachsous reverse primer: 5′-AAGTAGGAGGAGCGAGGTCC-3′. Animal culture and embryo collection Platynereis embryos were obtained from a breeding culture established in the Institut Jacques Monod (Paris), according to the protocol of Dorresteijn et al . [58] . Staging of the embryos was done according to Fischer et al . [59] The embryos were fixed using 4% paraformaldehyde in PBS+0.1% Tween20 and stored at −20 °C in 100% methanol. WMISH and immunohistochemistry Single nitro blue tetrazolium/5-bromo-4-chloro-3-indolyl phosphate (NBT/BCIP) WMISH were performed as follows. Embryos (previously stored in methanol) were rehydrated and washed in PBS. Digestion of the larval cuticle was done by incubating embryos during 1 min in a 100 μg ml −1 solution of proteinase K. Embryos were subsequently post-fixed in paraformaldehyde 4% for 20 min. Embryos were incubated overnight with RNA probes (marked with digoxigenin) in hybridization buffer (Torula RNA+heparine+formamide+sodium citrate buffer) at 65 °C, then washed in saline sodium citrate buffer and formamide at 65 °C. This was followed by a 1 h blocking in PBS+sheep serum, followed by an incubation with primary anti-digoxygenin-alkaline phosphatase antibody (Roche, 1:4,000) in PBS+sheep serum for 1 h. Embryos were washed in Tris-NaCl buffer pH7.5 and incubated in staining buffer (Tris-NaCl pH9.5+MgCl 2 ) for 10 min. Embryos were then incubated in staining buffer containing NBT/BCIP until a satisfactory staining was obtained. Stained embryos were washed first in Tris-NaCl buffer pH7.5, then in PBS and finally transferred in glycerol 87%. For antibody labelling, the same protocol as for the WMISH was used for embryo rehydratation, cuticle digestion and post-fixation. Embryos were blocked in PBS+sheep serum and then incubated for 1 h with the primary antibody in PBS+sheep serum. We used primary mouse anti-acetylated tubulin antibody (Sigma T7451; 1:500) and rabbit anti-phospho histone H3 antibody (Millipore 06-570, 1:100e). After several washes in PBS, embryos were blocked again in PBS+sheep serum and then incubated for 1 h with secondary antibodies in PBS+sheep serum. Secondary antibodies used were fluorescent anti-mouse IgG Alexa Fluor 488 or 555 conjugate (Invitrogen, 1:500). After several washes in PBS, the embryos were counterstained with Hoechst (1:1,000) and transferred in glycerol 87%. Cell proliferation and TUNEL assay Incorporation of embryos in EdU (200 mM) was done directly in sea water, for 30 min before fixation. Embryos were then fixed and stored at −20 °C in methanol. Labelling was done after rehydration, cuticle digestion and post-fixation, using the procedure described for WMISH. The labelling reaction was done according to the protocol of the Click-iT EdU kit (Molecular Probes). Embryos were then rinsed in PBS and counterstained with Hoechst (1:1,000). For TUNEL assays, after embryo rehydration, cuticle digestion and post-fixation, the terminal deoxynucleotide transferase reaction was performed following the protocol of the Click-iT TUNEL kit (Molecular Probes), with the following modification: embryos were left on ice during 1 h in the reaction cocktail before incubation of 1 h at 37 °C. Embryos used for positive control were incubated with DNAseI to generate DNA breaks (similar incubation, 1 h on ice followed by 1 h at 37 °C). Labelling was then performed following the protocol of the Click-iT TUNEL kit (Molecular Probes). For coupled WMISH, antibody staining and EdU labelling, the Clickt-iT EdU reaction was performed after NBT/BCIP WMISH and before antibody labelling. Small molecule inhibition Embryos were incubated during various time windows (see Results) in sea water containing endo-IWR-1 (Tocris Bioscience; 40 μM), PNU-74654 (Sigma-Aldrich; 5 μM), azakenpaullone (Sigma-Aldrich; 15 μM) or Y-27632 (Stemgent; 40 μM). Concentrations were on a test scale (from 10–40 μM for endo-IWR-1 and Y27632, from 1–25 μM for PNU-74654 and azakenpaullone). Stock solutions were 10 mM in 100% DMSO for endo-IWR-1, PNU-74654 and Y-27632; or 1 mM in 100% DMSO for azakenpaullone. Control embryos originating from the same batch were incubated in sea water containing 0.4% DMSO for endo-IWR-1 and Y27632, 0.05% DMSO for PNU-74654 and 1.5% DMSO for azakenpaullone. Cell counting Confocal images have been acquired on 12 control embryos and 12 embryos treated with endo-IWR-1 following a standardized procedure (50 slices, each 0.96 μM thick, posterior view). A region of interest corresponding to the neurectoderm has been delimited on these images using the ImageJ software. Samples have then been three-dimensionally reconstructed using the Imaris software (Bitplane) and cells have been counted using the three-dimensional spot tool of Imaris. Accession codes: Sequence data have been deposited in the GenBank/EMBL/DDBJ nucleotide database under accession codes HE858359 , HE858360 , HE858361 , HE858362 , HE858363 , HE858364 , HE858365 , HE858366 , HE858367 , HE858368 , HE858369 , HE858370 , HE858371 , HE858372 and HE858373 . How to cite this article: Demilly, A. et al . Involvement of the Wnt/β-catenin pathway in neurectoderm architecture in Platynereis dumerilii . Nat. Commun. 4:1915 doi: 10.1038/ncomms2915 (2013).